Prediction of extreme floods in the eastern Central Andes based on a complex networks approach Changing climatic conditions have led to a significant increase in the magnitude and frequency of extreme rainfall events in the Central Andes of South America. These events are spatially extensive and often result in substantial natural hazards for population, economy and ecology. Here we develop a general framework to predict extreme events by introducing the concept of network divergence on directed networks derived from a non-linear synchronization measure. We apply our method to real-time satellite-derived rainfall data and predict more than 60% (90% during El Niño conditions) of rainfall events above the 99th percentile in the Central Andes. In addition to the societal benefits of predicting natural hazards, our study reveals a linkage between polar and tropical regimes as the responsible mechanism: the interplay of northward migrating frontal systems and a low-level wind channel from the western Amazon to the subtropics. Prediction of extreme rainfall events and their impact on society are challenging tasks and rainfall occurrence in the eastern Central Andes (ECA) can only be understood in the broader context of the South American Monsoon System. A constant feature of the core monsoon season in South America (December through February, DJF) is the transport of moist air by low-level trade winds from the tropical Atlantic Ocean to the Amazon Basin along the Intertropical Convergence Zone [1] . However, the strength and direction of the subsequent moisture flow to the subtropics is subject to considerable variability: possible exit regions range from central Argentina to southeastern Brazil. A pronounced southward component towards the ECA is associated with the South American Low-Level Jet (SALLJ [1] , [2] ), and a southward extension thereof, the Chaco Jet [3] . These circulation regimes, which are partly controlled by the Northwestern Argentinean and the Chaco Low [3] , [4] , [5] , have been associated with increased precipitation in southeastern South America (SESA [6] ). Southward-directed anomalies of the large-scale moisture flow are also associated with enhanced rainfall in the ECA due to orographic lifting: increased moisture flux is forced to rise at the Andean mountain front and leads to pronounced orographic rainfall [7] , [8] . The cause of the circulation variability and the corresponding rainfall anomalies has not yet been identified in a way that sufficiently resolves the temporal order of events [9] , [10] , [11] , [12] . Since this is crucial for predicting associated extreme rainfall events, an early warning system for extreme rainfall in the ECA has been lacking. These events lead to severe infrastructural damage with large societal and economic ramifications: for instance in early 2007, natural hazards associated with intense rainfall events in the ECA affected more than 133,000 households and resulted in estimated costs of 443 million USD [13] . In this study, we provide all theoretical information necessary to forecast spatially extensive extreme rainfall at the ECA. For this purpose, we introduce the concept of network divergence, which is based on the non-linear synchronization measure Event Synchronization (ES) [14] , [15] , [16] , [17] and complex network theory. Recently, complex networks have attracted much attention for studying the spatial characteristics of temporal interrelations between climate time series [18] , [19] , [20] , [21] , [22] , [23] , [24] . The new measure network divergence introduced here is designed to assess the predictability of extreme events in significantly interrelated time series. We present and apply our new method with emphasis on extreme rainfall, but the methodology is more general and can be applied to a wide class of problems, ranging from climatic extreme event series to earthquakes, epileptic seizures or data from financial markets. Climatic mechanism During DJF, the spatial distribution of rainfall is strongly influenced by the interplay of the southward shift of the Intertropical Convergence Zone and the orographic barrier of the Andes ( Fig. 1a ), leading to enhanced precipitation at the eastern Andean slopes, along the South Atlantic Convergence Zone [25] , and in parts of SESA ( Fig. 1b ). There exist strong spatial gradients in the amount of rainfall accounted for during events above the 99th percentile ( Fig. 1c ). Most notably, very few extreme events (seven per season on average) account for more than 50% of total DJF rainfall in large parts of subtropical South America. We observe and corroborate earlier results [26] that in the ECA, frequency as well as magnitudes of extreme events in DJF have increased substantially during the past decades ( Fig. 1d , Supplementary Figs 1–3 ). 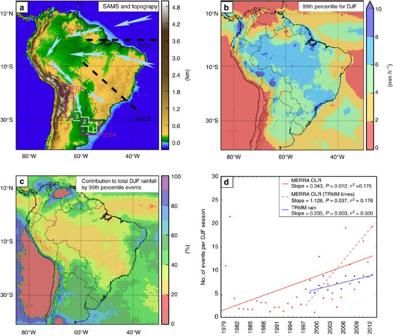Figure 1: Geographic and climatic setting. (a) Topography and simplified South American Monsoon System mechanisms. The boxes labelled 1 to 7 indicate the climatological propagation path of extreme events as revealed by the network analysis. (b) 99th percentile of hourly rainfall during DJF derived from TRMM 3B42V7 (ref.27in the spatial domain 85°W to 30°W and 40°S to 15°N, at a horizontal resolution of 0.25° × 0.25° and 3-hourly temporal resolution. (c) Fraction of total DJF rainfall accounted for by events above the 99th percentile. (d) Trend lines for the number of extreme events per DJF season averaged over boxes 6 and 7 ina: for TRMM rainfall (108 events in total, green solid line) for the period from 1998 to 2012 and MERRA outgoing longwave radiation (OLR29), for the period from 1979 to 2013 (252 events in total, red solid line) and for comparison for the period from 1998 to 2012 (red dashed line). Outgoing longwave radiation is used as a proxy for convective rainfall. Figure 1: Geographic and climatic setting. ( a ) Topography and simplified South American Monsoon System mechanisms. The boxes labelled 1 to 7 indicate the climatological propagation path of extreme events as revealed by the network analysis. ( b ) 99th percentile of hourly rainfall during DJF derived from TRMM 3B42V7 (ref. 27 in the spatial domain 85°W to 30°W and 40°S to 15°N, at a horizontal resolution of 0.25° × 0.25° and 3-hourly temporal resolution. ( c ) Fraction of total DJF rainfall accounted for by events above the 99th percentile. ( d ) Trend lines for the number of extreme events per DJF season averaged over boxes 6 and 7 in a : for TRMM rainfall (108 events in total, green solid line) for the period from 1998 to 2012 and MERRA outgoing longwave radiation (OLR [29] ), for the period from 1979 to 2013 (252 events in total, red solid line) and for comparison for the period from 1998 to 2012 (red dashed line). Outgoing longwave radiation is used as a proxy for convective rainfall. Full size image To estimate the dynamics and temporal order of extreme rainfall in South America, we computed network divergence for the satellite-derived and gauge-calibrated rainfall dataset TRMM 3B42V7 (ref. 27 ) ( Fig. 2a ). The NW-to-SE stretching source regions over the Amazon Basin and over the equatorial Brazilian Atlantic coast can be attributed to Amazonian squall lines [16] , [28] . Climatologically, the low-level flow from the Amazon towards the subtropics follows the band of sinks along the Bolivian Andes, which splits into two branches close to the Paraguayan border, corresponding to the SALLJ [2] and the Chaco Jet [3] , respectively. The most pronounced source region of the rainfall network is SESA, defined as the box ranging from 35°S to 30°S and 60°W to 53°W ( Fig. 1a ). To investigate where synchronized extreme events occur within 2 days after extreme events occurred in SESA, we calculated the spatially averaged ES from SESA to each grid cell ( S out (SESA), Fig. 2b ) and, for comparison, from each grid cell to SESA ( S in (SESA), Fig. 2c ). This analysis reveals that extreme events in SESA are followed by extreme events along a narrow band following the eastern Andean slopes up to western Bolivia ( Fig. 2b ), while they are only preceded by extreme events to the southwest ( Fig. 2c ). These observations are consistent with the results for S in (ECA), showing that synchronized extreme events in the ECA occur within 2 days after they occurred in SESA ( Supplementary Fig. 4 ). 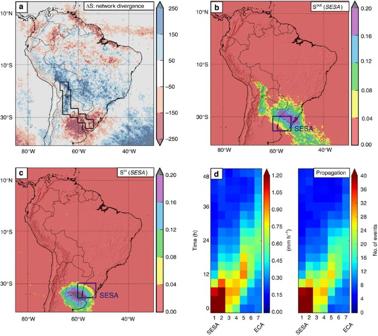Figure 2: Results of the network analysis and propagation of extreme rainfall from SESA to ECA. (a) Network divergence, defined as the difference of in-strength and out-strength at each grid cell,. Positive values indicate sinks of the directed and weighted network, which are interpreted as locations where synchronized extreme rainfall occurs within 2 days after it occurred at several other locations. On the other hand, negative values indicate sources, that is, locations where synchronized rainfall occurs within 2 days before it occurs at several other locations. The boxes labelled 1 to 7 are used for the tracking of extreme events shown ind. (b) Strength out of SESA,(SESA), which is the average Out-Strength restricted to SESA. Note in particular the high values along ECA. (c) Strength into SESA,(SESA), which is the average In-Strength restricted to SESA. Note in particular that there are no high values along ECA. (d) Temporal evolution of extreme rainfall events from SESA to ECA along the sequence of boxes indicated in (a). Composite rainfall amounts (left) and number of extreme events (right) in the respective boxes between SESA and ECA are displayed for propagation times and the subsequent 48 h. Each box has an edge length of 3° (~333 km), resulting in a total distance of ~2000, km. Figure 2: Results of the network analysis and propagation of extreme rainfall from SESA to ECA. ( a ) Network divergence, defined as the difference of in-strength and out-strength at each grid cell, . Positive values indicate sinks of the directed and weighted network, which are interpreted as locations where synchronized extreme rainfall occurs within 2 days after it occurred at several other locations. On the other hand, negative values indicate sources, that is, locations where synchronized rainfall occurs within 2 days before it occurs at several other locations. The boxes labelled 1 to 7 are used for the tracking of extreme events shown in d . ( b ) Strength out of SESA, (SESA), which is the average Out-Strength restricted to SESA. Note in particular the high values along ECA. ( c ) Strength into SESA, (SESA), which is the average In-Strength restricted to SESA. Note in particular that there are no high values along ECA. ( d ) Temporal evolution of extreme rainfall events from SESA to ECA along the sequence of boxes indicated in ( a ). Composite rainfall amounts (left) and number of extreme events (right) in the respective boxes between SESA and ECA are displayed for propagation times and the subsequent 48 h. Each box has an edge length of 3° (~333 km), resulting in a total distance of ~2000, km. Full size image For certain atmospheric conditions, extreme rainfall in SESA is synchronized with extreme rainfall in the ECA within the subsequent 2 days. Since ES identifies times with high synchronization between these regions, we can determine the corresponding atmospheric conditions by constructing composites of geopotential height and wind fields for these times. We use the following framework to identify times of high synchronization between SESA and ECA: We refer to 3-hourly time steps for which at least 15 grid cells in SESA (corresponding to an area of ~11,000 km 2 or 2% of the SESA area as depicted in Fig. 1a ) receive an extreme event as SESA times. This corresponds to time steps for which the number of extreme events at SESA is above the 60th percentile, computed on the set of time steps with at least one event. Furthermore, using the time series of synchronizations between SESA and ECA, we define SYNC times as time steps for which each grid cell in SESA receives an extreme event that synchronizes (within 2 days) with extreme events at more than four locations in the ECA. This corresponds to time steps for which the number of events at SESA that synchronize with one or more events at ECA is above the 80th percentile. Our results do not depend on small variations of the specific thresholds used to define SESA and SYNC times. SESA times that are also SYNC times will be called propagation times, while SESA times that are not SYNC times will be referred to as non-propagation times (see Table 1 ). For the 15 DJF seasons considered here, we obtain 502 propagation times occurring during 136 connected storm periods of maximal length of 3 days (that is, nine per DJF season), while there are 582 non-propagation times during 164 storm periods. During propagation times, extreme events propagate along the sequence of a roughly SE-NW oriented swath profile (white boxes in Figs 1a and 2a ) from SESA to ECA ( Fig. 2d ), that is, in the opposite direction of the low-level flow from the Amazon. Table 1 Different conditions used to determine the climatic mechanism and to formulate the forecast rule. Full size table For the purpose of recognizing the conditions under which extreme events in SESA synchronize with extreme events in the ECA, we construct composite anomalies relative to DJF climatology of geopotential height and wind fields both at 850 mb for propagation times and non-propagation times ( Fig. 3 ). Geopotential height and wind fields are derived from NASA’s Modern-Era Retrospective Analysis for Research and Applications (MERRA) dataset [29] . 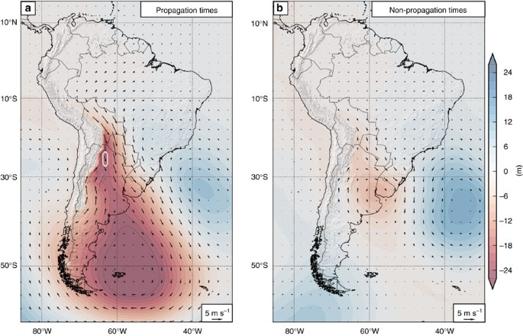Figure 3: Atmospheric conditions for propagation and non-propagation times. (a) Composite anomalies relative to DJF climatology of 850 mb geopotential height and wind fields from NASA’s Modern-Era Retrospective Analysis for Research and Applications (MERRA,29) for propagation times. Temporal resolution is 3-hourly, spatial resolution is 1.25° × 1.25°. The white polygon delineates the region over which the geopotential height anomalies are computed for the forecast rule. (b) The same composite anomalies as for (a), but for non-propagation times. Figure 3: Atmospheric conditions for propagation and non-propagation times. ( a ) Composite anomalies relative to DJF climatology of 850 mb geopotential height and wind fields from NASA’s Modern-Era Retrospective Analysis for Research and Applications (MERRA, [29] ) for propagation times. Temporal resolution is 3-hourly, spatial resolution is 1.25° × 1.25°. The white polygon delineates the region over which the geopotential height anomalies are computed for the forecast rule. ( b ) The same composite anomalies as for ( a ), but for non-propagation times. Full size image The composites identify northward propagating frontal systems and the associated low-pressure anomalies as common drivers of extreme rainfall in SESA and the establishment of a low-level wind channel from the Amazon to the subtropics: a low-pressure anomaly originating from Rossby-wave activity propagates northwards, led by a cold front causing abundant rainfall in SESA through the uplifting of warmer air masses [9] , [10] , [30] , [31] . When the frontal system propagates from SESA northeastward through the La Plata Basin in northeastern Argentina, the low-pressure anomaly extends to central Bolivia and merges with the Northwestern Argentinean Low [4] , [12] ( Fig. 3a ). This leads to the opening of a geostrophic wind channel along the resulting isobars that was previously blocked by the Andes Cordillera. This channel acts as a conveyor belt and transports warm and moist air from the Amazon Basin along the eastern slopes of the Andes and collides with the cold air carried by the frontal system. In combination with orographic lifting effects, this leads to extreme rainfall in the ECA within 2 days of the initial rainfall in SESA. The enhanced moisture flow to SESA after the initiation of rainfall can be assumed to be further stabilized by the release of latent heat [4] , [32] . With the cold front moving north, the flow will change its direction accordingly. A comparison with ref. 33 suggests that this climatic regime may be associated with Mesoscale Convective Systems [6] , which are formed over SESA and propagate upstream. A similar climatic regime has also been described in the context of so-called cold surges: northward incursions of cold air from midlatitudes [34] , [35] . Extreme event forecast Typically, rainfall events propagate from SESA to the ECA within the first day after the initial event in SESA ( Fig. 2d ), with an average speed of ~80 km h −1 . These results can be used to establish an operational early warning system of floods in the ECA. We employ the 3-hourly real-time satellite product TRMM 3B42V7 RT [27] for the time period from 2001 to 2013. To forecast extreme rainfall events in the ECA, we define prediction times as SESA times with a low-pressure anomaly in northwestern Argentina (geopotential height anomalies less than −10 m in white polygon in Fig. 3a ; this condition is abbreviated as GPH in Table 1 ). There are in total 649 such prediction times, occurring during 139 connected periods, resulting in an average of 10 such periods per season. The rainstorms associated with these events are likely to lead to severe floods and landslides downstream [13] , [36] because of their large spatial extent combined with little to no rainfall infiltration at high elevations: During the 2 days following prediction times, about 1/4 of each of the four boxes comprising ECA (boxes 4 to 7 in Fig. 1a ) receive an extreme event, corresponding to about 28,000 km 2 ( Supplementary Fig. 5 ). In particular, in the northern part of ECA (box 7 in Fig. 1 ), extreme events propagate to high elevations: in the northernmost box 7, at altitudes higher than 3,000 m above sea level, still about 60% (80% during positive El Niño Southern Oscillation (ENSO) phases) of all extreme events occur during prediction times ( Supplementary Figs 6 and 7 ). For the TRMM 3B42V7 RT dataset, more than 60% of all extreme events and of total DJF rainfall occur in the ECA during the 48 h following prediction times ( Supplementary Figs 8 and 9 ). During positive ENSO phases, they account for more than 90% of extreme rainfall events and more than 80% of total DJF rainfall in the northern parts of the ECA as well as on parts of the Bolivian Altiplano ( Supplementary Figs 10 and 11 ). To take into account the spatial extension of extreme rainfall, we formulate our forecast rule as follows: whenever the conditions of prediction times are fulfilled, there will be at least 100 events above the 99th percentile during the following 2 days in at least one of the ECA boxes (white boxes 4 to 7 in Fig. 2a ). Note that the corresponding average number of extreme events within such two-day periods is 50. To assess the skill of this simple forecast rule, we employ the Heidke Skill Score (HSS [37] ). This score yields HSS=0 for a uniformly random forecast and HSS=1 for a perfect forecast. For our forecast rule, we obtain HSS=0.47 when computed for all times during the DJF seasons between 2001 and 2013. We recall, however, that the considered climatic regime is only responsible for 60% of extreme events in the ECA. This implies that the remaining 40% can by construction not be predicted by our forecast rule, and the HSS is accordingly reduced. Moreover, the forecast skill certainly depends on the specific choice of the spatial boxes 4 to 7 and may change by adjusting their position. For positive ENSO conditions, we obtain HSS=0.57. The HSS is rather insensitive to variations of the condition on the number of extreme events in SESA and the exact geopotential height anomaly in northwestern Argentina, while it decreases rapidly for more events to be predicted in the ECA ( Supplementary Figs 12 and 13 ). We note that, while the mechanism responsible for these extreme rainfall events in the ECA was uncovered using network divergence, the conditions used for the forecast rule can be determined directly and with little computational efforts by spatially averaging rainfall and geopotential height data. We emphasize that we did not train the proposed forecast rule in the sense of parameter optimization. Instead, the rule is derived directly from the results of the network divergence analysis and we show that its forecast skill does not change rapidly when changing the conditions used to define prediction times. Our results provide all information necessary to implement an operational forecast system of extreme rainfall events in the ECA. It is very unlikely that previous state-of-the-art weather forecast models could predict these events: first, the propagation pattern only appears for very high event thresholds (97th percentile or higher, see Supplementary Fig. 14 ), and this ‘heavy tail’ of the rainfall distribution is not well implemented in current weather forecast models (see ref. 38 and citations therein). Second, for the regional climate model ETA, which is used at the Center for Weather Forecasting and Climate Research for operational weather forecast in South America, we compared the synchronization strength of SESA with the pattern found for TRMM and concluded that this model does not reproduce the propagation of extreme events from SESA to ECA ( Supplementary Fig. 15 ). Furthermore, while the climatological phenomenon of cold surges has already been described in other studies (by refs 34 , 35 ), only the usage of the high-spatiotemporal satellite product TRMM 3B42 allows to uncover the propagation of extreme events from SESA to ECA. This mechanism could not be found on the basis of reanalysis data such as the European Centre for Medium-Range Weather Forecasts Interim Reanalysis or NASA’s MERRA precipitation product ( Supplementary Fig. 15 ). In summary, applying network divergence to high-spatiotemporal resolution rainfall data identified a climatic mechanism that allows to predict more than 60% (90% during positive ENSO conditions) of rainfall events above the 99th percentile in the ECA from two conditions: preceding extreme rainfall at SESA and the presence of a low-pressure anomaly in northwestern Argentina. Data We employ the remote-sensing derived and gauge-calibrated rainfall data TRMM 3B42V7 (ref. 27 ) in the spatial domain 85°W to 30°W and 40°S to 15°N, at horizontal resolution of 0.25° × 0.25°, and 3-hourly temporal resolution for the time period from 1998 to 2012. To test our forecast rule, we use the (near) real-time satellite product TRMM 3B42V7 RT (ref. 27 ) with identical temporal and spatial resolutions for the time period from 2001 to 2013. Geopotential height and wind fields at 850 mb as well as Outgoing Longwave Radiation were obtained from NASA’s MERRA [29] . Extreme rainfall events are defined as times with rainfall above the 99th percentile of all DJF seasons, which results in 108 (94) 3-hourly events at each grid cell for the 15 (13)-year rainfall time series of the gauge-calibrated (real-time) version of TRMM 3B42V7. Event synchronization We employ the non-linear synchronization measure ES to assess the predictability of extreme events. It was modified on the basis of the original measure introduced in ref. 14 . For all pairs of grid cells i and j , we calculate the normalized number of events at j , which can be uniquely associated with subsequent events at i and vice versa within a time window of 2 (16 time steps) days: suppose we have two event series e i and e j containing the times of events at grid points i and j , each containing l extreme events. Consider two events and , with and 0 ≤ μ , ν ≤ l . In case, there occur several events in a row at the same location, only the first is considered as an event, weighted by the number of events in a row. Thus, for each event , there is a weight . To decide if the two events can be uniquely assigned to each other in a time-resolved manner, we compute for the dynamical delay In addition, we can introduce a filter by declaring minimum and maximum delays ( τ min , τ max ) between and , which enables us to analyse processes on different timescales. In this study, we chose τ min =0, and τ max =16 time steps of 3 h, corresponding to 2 days. We put if and and otherwise. Directed ES from e j to e i is then given as the normalized sum of this, resulting in the ES matrix ES . We emphasize that this measure does not assume temporal homogeneity between the event series because the possible delay between events is dynamical, contrary to the static delay in more traditional linear correlation analysis, which are usually based on calculating, for example, Pearson’s Correlation Coefficient at prescribed time lags (we refer to Supplementary Note 1 and Supplementary Fig. 16 for a detailed comparison between ES and lead-lag analysis using Pearson’s Correlation Coefficient). Furthermore, ES can be used to compute the average strength of synchronization of extreme rainfall between geographic regions such as SESA and ECA as a function of time. This will allow us to identify times of enhanced synchronization, which we use to determine the responsible atmospheric conditions and, thereby, to formulate a forecast rule for extreme rainfall in the ECA. Complex networks From all values of ES , a network is constructed by representing the strongest and most significant values of ES by directed and weighted network links. For two grid cells, a link points from the grid cell where rainfall events typically occur first to the grid cell where synchronized events occur within the subsequent 2 days. We assign the respective value of ES to the corresponding network link as a weight. Technically, the complex network’s adjacency matrix A is obtained by calculating the 98th percentile of all values of ES and then setting all values below to 0, such that the network will be weighted and directed with a link density of 2%. This particular link density is chosen such that all links correspond to significant ( P value <0.05) values of ES with respect to the null-hypothesis described in the following subsection. The strength of synchronizations into (out of) a grid cell is the sum of weights of all links pointing to (from) this grid cell, and to spatially resolve the temporal order of extreme events we introduce the network divergence Δ S ( Fig. 2a ), defined as the difference of in-strength S in and out-strength S out at each grid cell: Positive values of Δ S indicate sinks of the network: extreme events in these time series are preceded by extreme events in other time series; negative values indicate sources: extreme events there are followed by extreme events in other time series. In addition, we define the strength out of and into a region R ( Fig. 2a,b ): and where | R | denotes the number of grid cells contained in R . Thus, for example, would imply perfect synchronization from each grid cell in R to i : there would be a link from each grid cell in R to i and each of these links would have weight equal to 1. Significance testing The test of statistical significance of ES values is based on independent surrogates, which preserve the number of events as well as the block structure of subsequent events: From each original time series (48,400 in total), we construct surrogate time series by uniformly randomly distributing blocks of subsequent events. Next, we compute ES between all randomized time series and, from the histogram of all these values, determine P values for the original outcomes of ES. All network links correspond to values of ES which are significant at 0.05-confidence level. Prediction skill Given the separations between forecasted and observed events indicated in Table 2 , the HSS [37] is defined as Table 2 Contingency table used for computing the Heidke Skill Score. Full size table for a skill comparison versus randomness. Applying our forecast rule to the 3-hourly forecast dataset (TRMM 3B42V7 RT), we find the values summarized in Table 3 for the time period 2001 to 2013. These values result in HSS=0.47 for all years and HSS=0.57 for positive ENSO years. Table 3 The specific values of a, b, c and d used to compute the HSS of the forecast rule. Full size table How to cite this article: Boers, N. et al. Prediction of extreme floods in the eastern Central Andes based on a complex networks approach. Nat. Commun. 5:5199 doi: 10.1038/ncomms6199 (2014).